A highly abundant bacteriophage discovered in the unknown sequences of human faecal metagenomes Metagenomics, or sequencing of the genetic material from a complete microbial community, is a promising tool to discover novel microbes and viruses. Viral metagenomes typically contain many unknown sequences. Here we describe the discovery of a previously unidentified bacteriophage present in the majority of published human faecal metagenomes, which we refer to as crAssphage. Its ~97 kbp genome is six times more abundant in publicly available metagenomes than all other known phages together; it comprises up to 90% and 22% of all reads in virus-like particle (VLP)-derived metagenomes and total community metagenomes, respectively; and it totals 1.68% of all human faecal metagenomic sequencing reads in the public databases. The majority of crAssphage-encoded proteins match no known sequences in the database, which is why it was not detected before. Using a new co-occurrence profiling approach, we predict a Bacteroides host for this phage, consistent with Bacteroides -related protein homologues and a unique carbohydrate-binding domain encoded in the phage genome. In the past decade, metagenomic sequencing efforts have started to reveal the microbes inhabiting our planet [1] , [2] , [3] and our body [4] , [5] , [6] , [7] , [8] , [9] , [10] , [11] , [12] , [13] , [14] , [15] , [16] , [17] , including bacteria and viruses. The first snapshots of the bacterial microbiome in the human gut that were taken by using metagenomics revealed a high interindividual diversity and many unknown genes [14] . More recently, large scale sequencing efforts revealed that in fact, many people share a similar intestinal flora, regardless of whether these similarities are viewed as discrete enterotypes [15] or as gradients [18] . Endeavours including the Human Microbiome Project (HMP) [16] and MetaHIT [17] laid a baseline for the healthy human microbiome, enabling research laboratories around the world to anchor their work. Among the numerous breakthroughs in this field are the discovery of important functions for microbes in healthy individuals [14] , and the associations between specific members of our intestinal flora and unexpected diseases ranging from obesity [19] to cancer [20] . The viral community in our gut, also known as the human gut virome is dominated by bacteriophages (phages). Viral metagenomic studies have revealed that, in sharp contrast to the bacteria on which these phages depend for their replication, the viral sequences are mostly unknown, that is, they have no homologues in the database [4] , [5] , [6] , [7] , [8] , [9] , [10] , [11] , [12] , [13] . Moreover, gut viromes are thought to be highly individual specific as a result of the rapid sequence evolution of phages and the dynamic microbial ecosystem in the gut [4] , [5] , [6] . This leads to a virome with a vast, uncharted sequence space that is often referred to as biological ‘dark matter’ and provides an unprecedented opportunity for the discovery of novel viruses [21] . Virus discovery efforts increasingly employ metagenomics as a relatively unbiased tool to explore and chart the virosphere. Several studies have used metagenomic shotgun reads to assemble complete viral genomes, including phages [22] and viruses that infect humans [23] . In these studies, DNA may be derived from isolated virus-like particles (VLPs), but interestingly, DNA isolated from total community samples may also contain sequences of viral origin, estimates ranging up to 17% based on homology of the reads to known reference sequences [6] , [8] , [17] , [24] , [25] . Bypassing the need for sequence homology to identify specific phages, a recent study employed a search image based on a tetranucleotide usage profile to identify potential Bacteroides -like phages in published metagenomes [24] . While Bacteroides is one of the major bacterial taxa inhabiting our gut, only two phage genomes that infect this taxon were previously described [22] , [26] . In this previous study, a total of 85 contigs were identified that were potentially derived from Bacteroides -infecting phages [24] . The sequences were in the length order of known Bacteroides phage genomes, but the genome sequences were not closed. There are two important hurdles to overcome in metagenomic virus discovery efforts. First, the sequences derived from one viral genome need to be identified among the mixed metagenomic reads (‘binning’) and assembled. Second, the role of the assembled genome in the gut ecosystem needs to be unravelled. In the case of a phage, this starts with the identification of its bacterial or archaeal host. Here, we address both these issues by exploiting the idea that interacting sequences co-occur across samples. Co-occurrence analysis is a strong tool to identify functionally related entities. For example, correlation of gene presence/absence across genomes, also known as phylogenetic profiling has been exploited to predict functional relationships between genes [27] . Similarly, co-occurrence across metagenomic samples has been used to predict ecological interactions between bacterial species [28] , [29] . Recently, similarity in read depth profiles across metagenomes has been introduced to bin contigs derived from the same genome, allowing the assembly of draft genomes from rare bacteria in the microbial community. This approach relies on the availability of multiple similar metagenomes, such as time series samples [30] or metagenomes obtained after extracting DNA with different protocols [31] . Here, we re-analyse previously published viral metagenomes, isolated from human faeces of 12 different individuals. These subjects comprised four pairs of healthy female monozygotic twins and their mothers from four unrelated families [8] . By using cross-assembly [32] , we create depth profiles of cross-contigs across individuals to discover sequences that co-vary in abundance across these metagenomes. After separate assembly of one viral metagenome, we obtain an ~97 kbp circular genome sequence of a novel bacteriophage (crAssphage) that is highly abundant in publicly available metagenomes. Next, we exploit the same concept of co-occurrence profiling to predict the phage–host relationship, since we expect that phages can only thrive when their host species is present. We perform phage–host prediction by using co-occurrence in parallel with several independent phage–host prediction approaches, including homology searches and identification of CRISPR spacers for the in silico prediction of phage–host relationships, all of which consistently suggest a Bacteroides host for crAssphage. Metagenome assembly and binning of ubiquitous contigs Metagenomes, and especially viral metagenomes, are often characterized by a majority of unknown sequences that have no homologues in the database [21] . Assembly of the short, second generation sequencing reads into longer contigs may facilitate their annotation and interpretation. Depending on the sequence diversity of the underlying microbial community, their genome sizes, and sequencing statistics including depth and read length, metagenome assembly can yield short or longer contigs, comprising genome sequences with different degrees of fragmentation. Binning of contigs derived from the same genome followed by re-assembly of the reads associated to these contigs can greatly improve assembly statistics [31] . Several binning strategies are commonly used. First, contigs derived from the same genome may be identified if they are homologous to a known reference genome, although this approach seems less suitable for completely novel genomes. Second, information from mate-paired sequencing reads may be exploited for de novo binning, if available. Third, oligonucleotide usage (k-mer profile binning) is a de novo binning approach suitable for longer contigs >1,000 nt, but it is not robust for short contigs [33] . Moreover, genomes with similar k-mer usage cannot be distinguished. Fourth, a recently introduced depth profile binning approach allowed the assembly of near-complete draft genomes from metagenome data [30] , [31] . Combining different metagenomic data sets in a cross-assembly is a simple way to create an occurrence profile for contigs, where the number of reads from a metagenome that are assembled into a contig represents the occurrence of that contig in the metagenome. The cross-assembly programme crAss [32] generates such an occurrence profile for each contig. By normalizing for metagenome size, these occurrence profiles can be transformed into depth profiles for all contigs. Here, we generated a de novo cross-assembly of 1,584,658 metagenomic reads derived from faecal viral metagenomes from twelve different individuals [8] . The 7,584 resulting cross-contigs had an N50 value of 2,638 nucleotides, and one short contig, contig07548 contained reads from all 12 individuals, indicating that it was possibly derived from a ubiquitous viral entity. Next, we used depth profile binning as well as homology binning to identify other contigs that were likely derived from the same ubiquitous viral genome as contig07548. First, we calculated Spearman’s correlation scores between the depth profile of contig07548 across the 12 samples, and the profiles of all other contigs ( Supplementary Data 1 ). This resulted in many contigs with highly similar abundance patterns across the viral metagenomes ( Supplementary Data 1 and Supplementary Fig. 1 ), indicating that they had a similar occurrence in the original samples. Second, we performed a blastn [34] search (e-value <10 −10 ) against Genbank [35] , resulting in significant hits for 1,591 cross-contigs. The Genbank sequence that was most frequently identified as the top hit for a contig (214 times out of 7,584 contigs) was a clone in an unrelated human gut metagenome (Genbank PopSet identifier 259114965, see Methods). Although this sequence represents an unannotated clone and not a complete reference genome, these results strongly suggest that many of the assembled cross-contigs are actually derived from a single genome that was present in all the 12 personal viral metagenome data sets, hidden among the unknown reads. crAssphage genome assembly To investigate if the cross-contigs identified above were indeed derived from the same genome, we carefully re-assembled all the reads from one of the personal viral metagenomes. Because we expected the viral quasispecies to contain sequence heterogeneities, we used assembly settings that allowed such diversity to be collapsed (specifically, a short word length and a large bubble size, see Methods). We used the viral metagenome of Twin 1 from Family 2 (F2T1) for this assembly [8] , because most reads in the ubiquitous cross-contigs were derived from this metagenome ( Supplementary Data 1 ). This allowed us to construct a circular chromosome of 97,065 base pairs (bp) at an average depth of 230-fold in the F2T1 viral metagenomic sample ( Fig. 1 ). We named this phage ‘crAssphage’ after the cross-assembly programme originally used to discover it [32] . Although we used de novo assembly, the crAssphage genome aligned a total of 31 sequences from the unrelated human gut metagenome in Genbank mentioned above over 99.3% of its length (blastn e-value <10 −43 , four small gaps of 7–406 bp remained). Note that this was an unrelated metagenome sequenced by a different laboratory, yet the average aligned sequence identity was 97.4%. This illustrates the extensive evolutionary conservation of the crAssphage genome sequence between the intestines of unrelated human individuals. Due to the permissive assembly settings, the genome sequence is a consensus of the viral quasispecies population that occurs in the F2T1 personal viral metagenome, as is common in metagenome assemblies [36] . 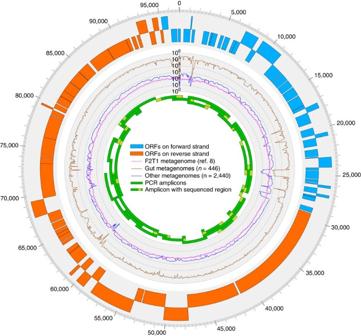Figure 1: Schematic representation of the circular crAssphage genome. The genome contains 80 ORFs that were predicted with Glimmer56trained onCaudovirales. The total coverage of each nucleotide in the F2T1 metagenome, and in all public metagenomes in MG-RAST49is indicated (466 human faecal and 2,440 other metagenomes, as determined by blastn mapping:⩾75 bp aligned with⩾95% identity, see Methods). Green bars indicate the 36 regions that were validated by long-range PCR (seeTable 2andSupplementary Table 1). Selected regions of several PCR amplicons (indicated as light green regions in the green bars) were sequenced by Sanger dideoxynucleotide sequencing to validate that the amplicons were indeed derived from the crAssphage genome (Supplementary Table 1). SeeSupplementary Fig. 6for the fully annotated figure. Figure 1: Schematic representation of the circular crAssphage genome. The genome contains 80 ORFs that were predicted with Glimmer [56] trained on Caudovirales . The total coverage of each nucleotide in the F2T1 metagenome, and in all public metagenomes in MG-RAST [49] is indicated (466 human faecal and 2,440 other metagenomes, as determined by blastn mapping: ⩾ 75 bp aligned with ⩾ 95% identity, see Methods). 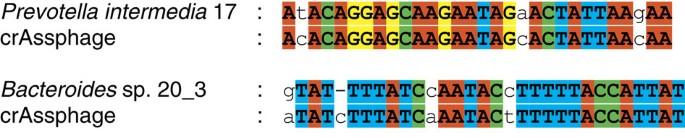Figure 2: CRISPR spacers similar to regions of the crAssphage genome. CRISPR spacers were identified in 2,773 complete bacterial genomes from Genbank, and in 404 genomes of intestinal isolates from HMP and MetaHIT. The CRISPR spacers that were most similar to the crAssphage genome were found inPrevotella intermedia17 (Genbank genomes) and inBacteroidessp. 20_3 (HMP and MetaHIT genomes). Conserved A, C, G, and T nucleotides are displayed in red, green, yellow and blue, respectively. Green bars indicate the 36 regions that were validated by long-range PCR (see Table 2 and Supplementary Table 1 ). Selected regions of several PCR amplicons (indicated as light green regions in the green bars) were sequenced by Sanger dideoxynucleotide sequencing to validate that the amplicons were indeed derived from the crAssphage genome ( Supplementary Table 1 ). See Supplementary Fig. 6 for the fully annotated figure. Full size image To validate that this sequence represented an existing chromosome in the original viral sample, we used the metagenomic sequences to design long-range PCR primers along the entire length of the genome and were able to amplify products of the expected size from the F2T1 sample ( Fig. 1 and Supplementary Fig. 2 , original viral preparation kindly provided by the authors [8] ) as well as from an unrelated faecal viral preparation (TSDC8.2, see Methods). A majority of the amplicons were partially sequenced by using Sanger sequencing to validate that they were indeed derived from the assembled crAssphage genome. As expected, higher sequence identity to the assembled crAssphage genome was observed between the Sanger sequencing traces derived from sample F2T1, than those from TSDC8.2 ( Supplementary Table 1 ). Encoded proteins Open reading frame (ORF) prediction identified 80 protein coding genes. They are largely co-oriented, being organized in two large blocks of ORFs encoded on the same strand ( Fig. 1 ). This genomic organization is typical of phage genomes, which frequently have a much larger fraction of their proteins encoded in sequential stretches on the same strand than bacterial genomes [37] . Functions could be annotated to a minority of the ORFs by a combination of homology searches in Genbank [35] and the Phage Annotation Tools and Methods database (PhAnToMe, http://www.phantome.org/ ), and domain searches using HHPred [38] ( Supplementary Data 2 ). Viral structural proteins were predicted using iVireons [39] . Among the annotated ORFs, a tentative clustering of functionally related proteins could be observed ( Supplementary Data 2 ). The HHPred search identified two hits to a Firmicute plasmid replication protein (RepL; PFam identifier PF05732 (ref. 40 )) in orf00050 and orf00102. Interestingly, these two ORFs occur close to the location where the coding directionality switches from the forward to the reverse strand. These conserved domains may facilitate the independent replication of the phage genome. Moreover, we identified several Bacteroidetes -associated carbohydrate-binding (BACON; PFam identifier PF13004 (ref. 41 )) domains present within orf00074 ( Supplementary Fig. 5 ). BACON is a recently identified domain mediating adherence to glycoproteins [41] . It has thus far only been found in Bacteroidetes genomes and in gut metagenomes, and was recently reported in another phage genome [7] . The homology-independent iVireons tool [39] predicted orf00074 to be a phage-structural protein (iVireons score 0.97, that is 85–88% accuracy). The presence of the BACON domain in a phage-structural protein might be explained by the recently proposed bacteriophage adherence to mucus model [42] . According to this model, phage adhere to the mucin glycoproteins composing the intestinal mucus layer through capsid-displayed carbohydrate-binding domains (such as the immunoglobulin-like fold or the BACON domain), facilitating more frequent interactions with the bacteria that the phage infects [42] . The homology searches did not provide strong clues as to the bacterial host of this phage. ORFs with homologues were all rooted deeply in the respective phylogenetic trees ( Supplementary Fig. 3 ). Moreover, top similarity of the ORFs was identified across multiple bacterial phyla ( Table 1 ) including Bacteroidetes (twelve hits, two of which were Bacteroidetes -infecting phages), Proteobacteria , (12 hits, 9 of which were Proteobacteria -infecting phages), Firmicutes (10 hits, 1 of which was a Firmicutes -infecting phage), Marinimicrobia (one hit), Actinobacteria and Cyanobacteria (each represented by one hit to a phage). Bacteriophages may range in their host specializations, some generalist phages infecting many, easily infectable bacteria [43] . Moreover, we suspect that the range of host taxa observed among the phage protein homologues reflects the sparseness of annotated sequence information available from gut phages. As a result, we mainly detected conserved or widespread phage proteins, including proteins involved in nucleic acid manipulation, and phage-structural proteins. Notably, the structural proteins are mostly associated with phage classes rather than with host classes. Finally, crAssphage rooted deeply in the phage proteomic tree [44] without close relatives ( Supplementary Fig. 4 ). Together, this shows that crAssphage represents a highly divergent genome sequence, with few clues for determining its role in the intestinal ecosystem. Table 1 CrAssphage ORFs with homology to known proteins or domains. Full size table Phage–host prediction Clustered regularly interspaced short palindromic repeats provide a form of acquired immunity to phages and plasmids in bacteria, consisting of multiple short direct repeats, and spacers derived from the encountered foreign DNA such as phage genomes [45] . Thus, CRISPR spacers have been used to recognize the phages that previously infected a certain bacterial genome [3] . To determine the bacterial host of crAssphage, we performed CRISPR searches [46] in 3,177 complete bacterial genomes. To provide a working immunity, CRISPR spacers should contain perfect matches to the viral genome, although recent studies have suggested that imperfect CRISPR matches could indicate recent interaction, facilitating rapid primed CRISPR adaptation [47] . In our analysis, none of the 93,276 identified CRISPR spacers had a perfect match to crAssphage. The most similar spacers were found in Prevotella intermedia 17 and in Bacteroides sp. 20_3, two intestinal species from the phylum Bacteroidetes ( Fig. 2 ). We also searched for sequence similarity of the 991 phage sequences previously identified by CRISPR targeting in human faecal metagenomes [48] (blastn, e-value ≤10), but no matches were found between these sequences and the crAssphage genome. Figure 2: CRISPR spacers similar to regions of the crAssphage genome. CRISPR spacers were identified in 2,773 complete bacterial genomes from Genbank, and in 404 genomes of intestinal isolates from HMP and MetaHIT. The CRISPR spacers that were most similar to the crAssphage genome were found in Prevotella intermedia 17 (Genbank genomes) and in Bacteroides sp. 20_3 (HMP and MetaHIT genomes). Conserved A, C, G, and T nucleotides are displayed in red, green, yellow and blue, respectively. Full size image Next, we attempted to link crAssphage to a bacterial host by using co-occurrence profiling. Because phages can only thrive in an environment if their cellular host is present, we expected the occurrence of crAssphage and its host to show a correlated pattern, similar to the correlations between the depth profiles of contigs derived from the same genome. Thus, we compared the depth profile of the crAssphage genome and of 404 intestinal bacterial strains forming potential hosts, across an expanded data set of 151 faecal community shotgun metagenomes from the HMP [16] (see Supplementary Data 3 ). These metagenomes contained both viral and bacterial sequences. We calculated Spearman's correlation values between all depth profiles and created a co-occurrence cladogram to identify which bacterial depth profiles clustered with that of crAssphage. As shown in Fig. 3 , crAssphage clusters deep within a group of Bacteroidetes genomes, suggesting one of the Bacteroides species as the most likely host. Similarly, two Bacteroides phages [22] , [26] that we included as positive controls also cluster among Bacteroidetes , although they recruited only a small fraction of metagenomic reads compared with crAssphage (104,076,280; 13,770; and 12,852 reads for crAssphage, B40-8 and B124-14, respectively). 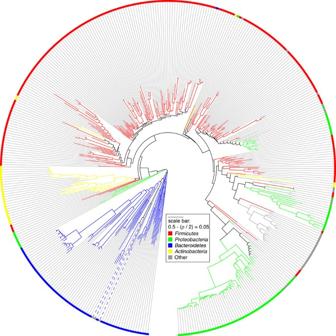Figure 3: Phage–host prediction based on co-occurrence across metagenomes. Unrooted co-occurrence cladogram of correlated depth profiles across 151 HMP faecal metagenomes16of the crAssphage, two knownBacteroides fragilis-infecting phages22,26, and 404 potential hosts. Colours indicate bacterial phyla. The phages are indicated with blue dashed lines. SeeSupplementary Fig. 7for the fully annotated figure. Figure 3: Phage–host prediction based on co-occurrence across metagenomes. Unrooted co-occurrence cladogram of correlated depth profiles across 151 HMP faecal metagenomes [16] of the crAssphage, two known Bacteroides fragilis -infecting phages [22] , [26] , and 404 potential hosts. Colours indicate bacterial phyla. The phages are indicated with blue dashed lines. See Supplementary Fig. 7 for the fully annotated figure. Full size image A recent study that identified Bacteroides phages by using a tetranucleotide search image identified 85 sequences of >10 kbp in size in published human faecal metagenomes [24] . None of these 85 sequences matched crAssphage in a homology search (blastn, e-value ≤10), while the data sets that were scanned for that previous study [24] , in fact contained 11 sequences >10 kbp and 72 sequences in total that were homologous to crAssphage, with a combined length of 408 kbp (results not shown). This emphasizes the uniqueness of the crAssphage genome both in terms of the sequence and in terms of its nucleotide-usage profile. Finally, plaque assays performed with phages from independent faecal isolates gave no additional insights (see Methods). None of the plaques that were observed on potential Bacteroides host strains tested positive when using crAssphage-specific PCR primers. Ubiquity of crAssphage in public metagenomes Next, we determined the ubiquity of the crAssphage sequence in all 2,944 publicly available DNA shotgun metagenomes in the MG-RAST database [49] , and compared it with previously known phages. These public metagenomes were sampled from a range of microbial environments, and were not limited to the human gut. To do this, we created a database consisting of 1,193 phage genomes including crAssphage and all complete phage genomes in the PhAnToMe database, and used this to align the public metagenomic reads (blastn, ⩾ 75 bp aligned, ⩾ 95% identity, ambiguously aligned reads were discarded). We detected reads that uniquely aligned to crAssphage in 940 of these metagenomes, including both total community metagenomes and viral metagenomes, among which were 342 of the 466 faecal metagenomes (73%). Previous reports have estimated that total community samples may also contain sequences of viral origin, estimates ranging up to 17% (refs 6 , 8 , 17 , 24 , 25 ). Here, we observed that the crAssphage genome accommodated up to 90% of the sequencing reads in the faecal viral (that is, VLP-derived) metagenomes from the twin study that we used as a starting point [8] ; up to 24% of the reads in an unrelated faecal viral metagenome from Korea [13] ; and up to 22% of the reads in total faecal community metagenomes from USA [16] ( Supplementary Data 4 ). Across all the metagenomes, 235.8 million reads aligned uniquely to crAssphage. Almost all these hits (235.5 million or 99.9%) were derived from human gut metagenomes, comprising 1.68% of all the reads in the metagenomes that were annotated as being derived from human faeces. Thus, crAssphage is significantly more abundant in human faeces than in other environments (one-tailed Kolmogorov–Smirnov test, P <2.2e −16 ). Based on this analysis, crAssphage is by far the most abundant, and one of the most ubiquitous bacteriophages in the publicly available metagenomes ( Fig. 4 and Supplementary Data 5 ). 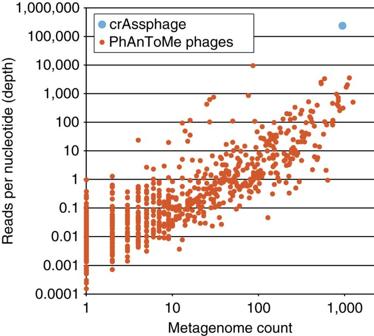Figure 4: Abundance ubiquity plot of phage genomes in public metagenomes. Reads from 2,944 publicly available shotgun metagenomes49were aligned to a database of 1,193 phage genomes (see Methods). The average depth of aligned reads per nucleotide of the phage genome (abundance) is plotted against the number of metagenomes it is found in (ubiquity). SeeSupplementary Data 5for details. Figure 4: Abundance ubiquity plot of phage genomes in public metagenomes. Reads from 2,944 publicly available shotgun metagenomes [49] were aligned to a database of 1,193 phage genomes (see Methods). The average depth of aligned reads per nucleotide of the phage genome (abundance) is plotted against the number of metagenomes it is found in (ubiquity). See Supplementary Data 5 for details. Full size image The read depth or recruitment profile of these reads along the crAssphage genome was stable in most of the public metagenomes ( Fig. 5 ), although several conspicuous gaps remained, that were apparent in many of the public metagenomes (indicated with arrowheads at the top of Fig. 5 ). Similar recruitment gaps have recently been observed in marine bacteriophages [50] , and have been suggested to result from a Constant-Diversity or Red Queen dynamics. Dubbed ‘metaviromic islands’, the rare or divergent regions, may contain genes that are under positive evolutionary selection, including host recognition and other proteins [50] . Two such ORFs on the crAssphage genome, orf00039 and orf00050, encode proteins with homology to an endonuclease and a plasmid replication protein, respectively. 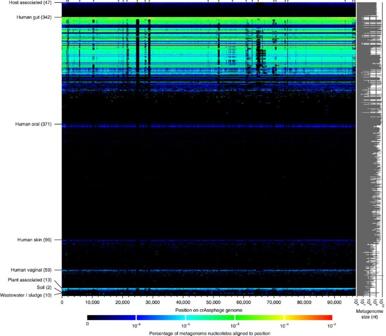Figure 5: Normalized coverage plot of the crAssphage genome in 940 public metagenomes. Rows are metagenomes, with the sequence volume in nucleotides indicated to the right (seeSupplementary Data 4for the order and detailed annotations of the metagenomes). Thexaxis of the heat map displays the 97,065 bp length of the crAssphage genome sequence. The colour bar indicates the percentage of nucleotides in each metagenome that aligns to each position. Black arrowheads at the top of the figure indicate metaviromic islands50. Details are available inSupplementary Data 4. Note that some of the metagenomes at the bottom of the plot that are annotated as ‘Plant-associated’ are also faecal metagenomes69. Figure 5: Normalized coverage plot of the crAssphage genome in 940 public metagenomes. Rows are metagenomes, with the sequence volume in nucleotides indicated to the right (see Supplementary Data 4 for the order and detailed annotations of the metagenomes). The x axis of the heat map displays the 97,065 bp length of the crAssphage genome sequence. The colour bar indicates the percentage of nucleotides in each metagenome that aligns to each position. Black arrowheads at the top of the figure indicate metaviromic islands [50] . Details are available in Supplementary Data 4 . Note that some of the metagenomes at the bottom of the plot that are annotated as ‘Plant-associated’ are also faecal metagenomes [69] . Full size image Many studies in the relatively young field of metagenomics aim to characterize environments in terms of the taxa and functions that are encoded on their communal genomes, or metagenomes. To do this, environmental shotgun sequencing reads are aligned to a reference database of annotated sequences using fast algorithms and intelligent shortcuts [49] , but this approach may leave a large fraction of the reads unannotated. Viruses are especially notorious in this respect. Being both under-sampled and rapidly evolving [21] , it has been suggested that the unknown fraction of metagenomes is enriched for viral sequences [51] . These sequences may either be disregarded altogether, or reported in a pie chart as a slice labelled ‘unknown’, but either way they represent a sizeable elephant in the room. Everyone agrees the unknowns may be important, yet they are commonly ignored. Here, we report the assembly of an ~97 kbp circular sequence from a previously published faecal viral metagenome. Our results strongly suggest that this sequence represents a phage genome that is highly divergent from the known phages currently present in the databases. First, the genome is highly abundant in some viral metagenomes that have been size- and density-filtered for VLPs, such as the F2T1 viral metagenome used to assemble it [8] . Second, the ORFs encoded on the genome show similarity to bacteriophage and bacterial proteins ( Supplementary Data 2 ). Although more than two thirds of the ORFs have no inferable function, we observe several functions that are typical of bacteriophages. Specifically, functions for DNA manipulation, replication and phage-structural proteins are encoded, while there is a distinct lack of any conserved bacterial or archaeal metabolic genes. Moreover, we observe a pattern of modularity among these functions. Third, the coding structure of the ORFs is typical of a phage genome. While the ORFs encoded on the crAssphage genome change strand directionality at two positions, the ORFs encoded on bacterial genomes change strand directionality much more frequently [37] . Fourth, although we did not find any transfer RNA genes (either prokaryotic or eukaryotic) in the genome sequence, the plethora of putative prokaryotic promoter patterns pillars the premise that this is a prokaryotic phage. Finally, we detected this genome in many metagenomes sequenced by different laboratories around the world, derived from different samples and sequenced using different sequencing technologies ( Supplementary Data 4 ). This limits the possibility that the sequence is derived from contamination of reagents. In this study, we exploited co-occurrence profiles across metagenomes in two ways to predict associations between sequence elements. First, we created cross-contigs by assembling the metagenomic reads from 12 personal viral metagenomes, and analysed their depth profiles using crAss [32] . These depth profiles were highly similar for the majority of the ubiquitous cross-contigs, suggesting that they were derived from the same genome ( Supplementary Data 1 ). This analysis also identified F2T1 as the person with the highest read depth for these ubiquitous contigs. Using this information, we then assembled the circular crAssphage genome from the F2T1 data set. By assembling only one metagenome, we minimized the heterogeneity in the assembled genome sequence. The genome assembly was validated with long-range PCR and Sanger dideoxynucleotide sequencing of several regions in two independent samples. We note that the presented genome sequence should be interpreted as a metapopulation consensus genome of the viral quasispecies that occurs in the sample [36] , where some sequence diversity remains. For example, this can be observed in the sequencing results of the PCR products, where higher sequence identity to the crAssphage genome is observed in the traces derived from the original sample, F2T1 than in the unrelated sample TSDC8.2, although some mutations relative to the assembled sequence still remain, even in F2T1 ( Supplementary Table 1 ). Second, we used co-occurrence profiling of the newly identified phage genome with 404 potential hosts across 151 faecal shotgun metagenomes from the HMP. These total community metagenomes contained bacterial reads (the potential hosts) as well as viral reads (for example, crAssphage). As a result, the occurrence profiles in our analysis contain the same data sets, precluding any spurious correlations due to differences in the sampling or sequencing protocol. Here, we have used the non-parametric Spearman rank correlation to determine links between the phage and its host. We note that other correlation measures or a combination thereof might also be appropriate [29] . Moreover, the correlative associations may be indirect. Although our approach could not specify the host to the level of species due to low correlation scores of crAssphage with the individual Bacteroidetes genomes, the clustering with this group was consistent with the other two Bacteroides phages ( Fig. 3 ). Moreover, this host prediction is in line with the unique Bacteroidetes -associated BACON domain [41] , the 12 annotated homologues in the phylum Bacteroidetes ( Table 1 ) and the two most similar CRISPR spacers ( Fig. 2 ). We are currently integrating these and other signals into a bioinformatic phage–host prediction framework to facilitate this important first step towards identifying the role of newly identified phages in the microbial ecosystem. Although phages and the associated kill-the-winner dynamics may result in a loss of correlation between the occurrence patterns of phages and their hosts, we postulate that this process acts at the level of strains, or even sub-strain types diverging only at the level of, for example, their surface proteins. While one bacterial strain may be killed by expansion of a specific cognate phage, closely related bacteria may still be present in those same metagenomes because they will have similar niche preferences. This is also supported by the apparent constant-diversity (also known as Red Queen) dynamics acting on only a few of the ORFs, that is, those that under-recruit reads from public metagenomes and are observed as metaviromic islands [50] ( Fig. 5 ). To summarize, here we identified and validated the ~97 kbp genome sequence of a novel bacteriophage, crAssphage. We show that its genome sequence is highly abundant and ubiquitous in publicly available metagenomes, and predominantly occurs in human faeces. This observation argues against the common view that the intestinal virome is unique to each individual, and suggests that some phages might be highly conserved in people around the world. Notably, little congruency was originally observed between the intestinal bacterial microbiota of different individuals [14] , whereas many people in fact share a similar intestinal flora [15] , [18] . Abundant phages and other mobile elements have previously been observed in metagenomes from the ocean [52] and the human gut [5] , [6] , [8] , [22] , [24] , [48] . However, most studies rely on aligning sequencing reads to a reference database for identifying phage sequences, ignoring the sometimes abundant unknowns. The observations presented here suggest that ignoring the unknown sequences in viral metagenomes may lead to an overestimation of the diversity in the human gut virome. Highly abundant, ubiquitous and conserved bacteriophages may remain hidden in the unknown fraction of metagenomes. Metagenomic sequencing data Metagenomic sequencing reads from human faecal viral metagenomes of four female twin pairs and their mothers [8] were downloaded from the NCBI Short Read Archive (accession number SRA012183 ). Because the original authors showed that the intrapersonal diversity was low, we combined metagenomes for each individual, resulting in 12 personal faecal viral metagenomes. Total shotgun metagenomes from human faeces, including both viral and bacterial sequences, were downloaded from HMP (151 Faecal Illumina WGS Reads and Assemblies HMIWGS/HMASM http://www.hmpdacc.org/HMASM/ , the accession numbers are listed in Supplementary Data 3 ). Assembly An initial metagenomic cross-assembly of the twelve combined faecal viral metagenomes was constructed by using gsAssembler [53] 2.6 ( ⩾ 65 nt overlap, ⩾ 98% identity) yielding 7,584 cross-contigs as identified with crass [32] version 1.2. By examining this cross-assembly, we discovered that many of these contigs had highly correlated depth profiles ( Supplementary Data 1 ) and were homologous to a few long clones from a metagenome in Genbank with the PopSet identifier 259114965, suggesting that they were derived from the same genome. As the F2T1 viral metagenome contributed the most reads within these contigs, all the reads from this metagenome were re-assembled de novo with CLC Genomics Workbench 6.0.4 (word size: 35, bubble size: 1,000), yielding three contigs with similarly high depth (lengths 64,230; 31,634; and 1,269 bp) that overlapped, allowing them to be merged into a circular genome of 97,065 bp with an average per base depth of 230-fold. This crAssphage genome sequence was deposited in Genbank with the identifier JQ995537. Primer design To validate the crAssphage genome sequence, we designed 24 primer pairs covering the entire genome sequence ( Table 2 ). Genome-wide primer design using jPCR [54] was supplemented with a conservation analysis of the sequence in the 12 personal viral metagenomes to ensure they matched within conserved genomic regions. The regions selected for amplification were between 498 bp and 18,342 bp in length ( Supplementary Fig. 2 ). Table 2 PCR primer pairs designed to validate the crAssphage genome sequence. Full size table Long-range PCR To validate the genome assembly of crAssphage, we obtained the original F2T1.2 sample of faecal viral DNA from the authors [8] (sample identifier: TS4.2). Moreover, an independent faecal viral sample was also included, obtained from a healthy adult monozygotic twin as part of a human gut microbiome survey [55] (sample identifier: TSDC8.2). The sample was processed for isolation of VLP-associated DNA as described [8] . The PCR was performed using the Thermo Scientific Hi-Fidelity Extensor Long-Range PCR Enzyme kit with 9 μl of the 2 × mix and 14 μl of water per reaction (Cat. No. AB-0792/A and AB-0720/B). A touchdown method was used for the PCR cycling conditions to account for differing melting temperatures of the primers. PCR cycling conditions were as follows: (1) denaturation at 95 °C for 2 min; (2) denaturation at 95 °C for 10 s; (3) annealing at 58 °C for 30 s; touchdown at −0.5 °C; (4) extension at 68 °C for 6.5 or 10 min; (5) repeat steps 2–4 thirty times; 6) final elongation at 68 °C for 10 or 14 min; store samples at 4 °C until further use. Extension times were adjusted for the expected product size, for example, for products of primer pair F3R3 with expected size 5.4 kbp, the extension time was 6.5 min. A 12 μl aliquot of PCR products was run on a 0.6 or 0.7% agarose gel for PCR products of 2–7 kbp and >8 kbp, respectively. A GeneRuler 1 kbp DNA ladder (Thermo Scientific) was used for comparison of all PCR products under ultraviolet luminescence. Proteins and annotation ORFs were predicted by using Glimmer [56] 3.02, that was trained with all Caudovirales genomes in the PhAnToMe database ( http://www.phantome.org ). ORF homologues were identified by using blastx [57] 2.2.27+ searches against the Genbank nr database [35] with an e-value cutoff of 0.01 ( Supplementary Data 2 ). After aligning ORFs with at least three homologues by using Clustal Omega [58] 1.1.0, maximum likelihood phylogenetic trees were created as described [59] . To identify more distant homologues, ORFs were queried by DeltaBLAST [60] against the Caudivirales subset of Genbank (NCBI taxonomy identifiers 28883 and 102294) with an e-value cutoff of 0.01. Moreover, ORFs were queried by HHPred [38] against the pdb70, scop70, CDD, InterPro, PfamA/PfamB, SMART, PANTHER, TIGRFAMs, PIRSF, SUPERFAMILY, CATH/Gene3D, and COG/KOG databases. These results are included in Supplementary Data 2 . We tested if ORFs were likely structural phage proteins by using iVireons [39] . Transmembrane helices were predicted by using HMMTOP [61] . To identify the BACON domain [41] , the crAssphage genome and all 1,192 complete viral genomes in the PhAnToMe database were scanned with GeneWise2 (ref. 62 ) which allows nucleotide sequence searches against the Pfam database of protein-based hidden Markov models [40] . The only hits to the BACON domain within these 1,193 viral genomes were eight hits that were all located within crAssphage orf00074 ( Supplementary Fig. 5 ). Although the seven of the associated bit scores are lower than the cutoff of 25 that has been considered significant [63] , it should be noted that these eight hits lie within one protein, orf00074, and were the only BACON domains found in any of the screened genomes. Phage proteomic tree The phage proteomic tree was constructed as described [44] . Briefly, families of related proteins identified by using blastp [34] were aligned, and PROTDIST [64] alignment scores combined to provide a pairwise distance between all genomes, compensating for missing proteins and the protein lengths in each family. A neighbor-joining tree was constructed from the distance matrix [64] . The phage proteomic tree shows that while the known Bacteroides phages B124-14 (ref. 22 ) and B40-8 (ref. 26 ) are closely related, crAssphage is only distantly related to other viruses ( Supplementary Fig. 4 ). Phage–host prediction by co-occurrence Occurrence of the crAssphage genome was measured in 151 complete faecal community metagenomes from the HMP by aligning the metagenomic sequencing reads with Bowtie [65] 0.12.8. Similarly, the occurrence pattern was measured of two positive controls, the known Bacteroides fragilis -infecting phages B124-14 (NC_016770.1 (ref. 22 )) and B40-8 (NC_011222.1 (ref. 26 )). Read aligning yielded highly similar hits (~3.2±1.9 mismatches). Finally, reads were also aligned to 404 genomes of faecal isolates including the HMP reference genomes from the gastrointestinal tract ( n =372, downloaded on 19 February 2013 from [66] http://www.hmpdacc.org/HMRGD/ ) and the MetaHIT draft sequences ( n =32, downloaded on 19 February 2013 from http://www.sanger.ac.uk/resources/downloads/bacteria/metahit/ ). After normalization, a distance score between all pairs of depth profiles was calculated as 0.5−( ρ /2), where ρ is the Spearman rank correlation between the depth profiles. The symmetrical distance matrix was converted to a co-occurrence cladogram by using BioNJ [68] ( Fig. 3 ). Clustering with the phages separately did not change their association to the Bacteroidetes cluster. Testing for crAssphage in CRISPR spacers Using pilercr v1.06 (ref. 47 ), we screened 2,773 complete prokaryotic genomes from Genbank [35] and 404 faecal isolates (above), identifying 79,977 and 13,299 CRISPR spacers, respectively. All spacers were queried by using blastn 2.2.27+ with short query parameters [57] against the crAssphage genome. The best global hits from either collection of genomes (that is along the complete spacer length) are displayed in Fig. 2 . Both these spacers match genomes from the class Bacteriodetes . Plaque assays We attempted to isolate crAssphage by isolating Bacteroides -specific phages from faecal phage lysates using an adapted plaque assay method [68] . To do this, we obtained 10 phage lysates from faecal samples. A quantity of 1 ml sodium magnesium (SM) buffer was added to faecal sample and vortexed on high for 1 h. SM buffer contained (per 500 ml): 2.9 g NaCl (Fisher Scientific, Waltham, MA), 1 g MgSO 4 7H 2 O (Fisher Scientific) and 25 ml of 1 M Tris–HCl pH 7.4 (Sigma-Aldrich, St Louis, MO). Samples were centrifuged for 4 min at 12,000 r.p.m. (revolutions per minute) (that is, 13.4 relative centrifugal force, r.c.f.) and the supernatant transferred to a clean tube. A quantity of 50 μl ml −1 of chloroform (Fisher Scientific) was introduced to the supernatant to arrest growth, vortexed briefly and incubated at 4 °C for 20 min. Following cold incubation, samples were centrifuged for 10 min at 4,000 r.p.m. (that is, 1.5 r.c.f. ), supernatant transferred to a clean tube and 15 μl of 100 units ml −1 DNase (Fisher Scientific) added. Samples were incubated at 35 °C for 1 h and subsequently incubated at 65 °C for 15 min. To separate viral-like particles (VLPs), remaining samples were passed through a 0.45 μm filter (Millipore Corporation, Billerica, MA) attached to a 3 ml syringe (Becton, Dickinson and Company, Sparks, MD). The resulting lysate was topped with additional SM buffer plus 16 mM MgSO 4 to reach a volume of 1 ml and stored at 4 °C. Two gut-associated Bacteroides strains were tested: the annotated host of the known Bacteroides phages B124-14 (ref. 22 ) and B40-8 (ref. 26 ), Bacteroides fragilis ; and B. thetaiotaomicron (stocks kindly provided by San Diego State University Microbiology Department, San Diego CA; SDSU-MD accession numbers 939 and 906, respectively). Phages were isolated using the adapted most probable number method [68] . 2 × Bacteorides phage recovery medium was incubated with a 1:1 mixture of host and phage lysate for 24 h at 37 °C. Following incubation, the incubated medium was subjected to chloroform at 50 μl ml −1 of broth to arrest any living host cells. Supernatant of the various conditions was spotted atop a fresh lawn of host on Bacteorides phage recovery medium agar plates. Plates were placed into a GasPak (BBL) jar and incubated at 37 °C for 16 h. Plaques appeared, and 10 pools of 10 plaques each were selected. DNA was extracted and PCR performed using the primer pairs F4R4, F4R6 and F23R23 as above ( Table 2 ). Although these primer pairs successfully amplified regions of the crAssphage genome from the faecal samples F2T1 and TSDC8.2 ( Supplementary Table 1 ), no bands were observed after application of the same primer pairs to the plaque pools, indicating that these plaques were probably caused by other Bacteroides -infecting phages. Phages in metagenomes To determine the prevalence of the crAssphage genome across different environments, we downloaded sequencing reads from all 2,944 publicly available shotgun metagenomes available in the MG-RAST database [49] . A database of 1,193 phage genomes was created by adding crAssphage to all complete phage genomes from PhAnToMe ( http://www.phantome.org ). A blastn [57] 2.2.27+ search of every metagenomic read versus the phage genome database was performed, and hits were considered if they had at least 95% identity over an aligned length of 75 bp. Ambiguously aligned reads were discarded. How to cite this article : Dutilh, B. E. et al . Unknown sequences in faecal metagenomes reveal a widely distributed and highly abundant bacteriophage. Nat. Commun. 5:4498 doi: 10.1038/ncomms5498 (2014). Accession codes : The crAssphage genome sequence was deposited in the Genbank Nucleotide sequence database with accession code JQ995537 . Sanger sequenced regions of the PCR products from F2T1 and TSDC8.2 (indicated by the light green regions of the green bands of Fig. 1 ) were deposited in the Genbank nucleotide sequence database with accession codes KM000086 to KM000121 (see Supplementary Table 1 ).